Quantification of plasma HIV RNA using chemically engineered peptide nucleic acids The remarkable stability of peptide nucleic acids (PNAs) towards enzymatic degradation makes this class of molecules ideal to develop as part of a diagnostic device. Here we report the development of chemically engineered PNAs for the quantitative detection of HIV RNA at clinically relevant levels that are competitive with current PCR-based assays. Using a sandwich hybridization approach, chemical groups were systematically introduced into a surface PNA probe and a reporter PNA probe to achieve quantitative detection for HIV RNA as low as 20 copies per millilitre of plasma. For the surface PNA probe, four cyclopentane groups were incorporated to promote stronger binding to the target HIV RNA compared with PNA without the cyclopentanes. For the reporter PNA probe, 25 biotin groups were attached to promote strong signal amplification after binding to the target HIV RNA. These general approaches to engineer PNA probes may be used to detect other RNA target sequences. Diagnostic testing of HIV in both infected and non-infected patients is crucial to control the disease within the global population [1] . Moving such tests closer to the point-of-care (POC) for a patient helps doctors to quickly discern infection status and select the proper antiretroviral medication [2] . Obtaining this information more quickly and accurately promotes a test-and-treat strategy that has known benefits to limit spread of the virus [3] . HIV tests performed at the POC are typically antibody based, qualitative and require some type of follow-up testing to confirm infection [4] , [5] , [6] , [7] , [8] , [9] . Despite the popularity of antibody-based tests, nucleic acid testing (NAT) for HIV RNA continues to be the ultimate standard to confirm an infection and it is also the only method to quantify the viral load within infected patients [10] , [11] . Plasma HIV RNA levels correlate very well with the acute phase of infection, when the virus is most likely to be transmitted, and increases in viral load signal when the virus has developed resistance to a particular antiretroviral therapy [12] . Despite the benefits of tracking plasma HIV RNA in patients, there is no standard nucleic acid-based test for HIV that can be used at a patient’s POC (ref. 13 ) and only about one-third of all public health laboratories in the US are equipped to perform NAT for HIV RNA [14] . There are even fewer public health facilities in developing countries that test for HIV RNA [15] . The lack of testing for HIV RNA reflects the complications of using reverse transcription-PCR (RT-PCR), the most common method to detect and quantify RNA [16] , [17] , [18] . The typical cost, instrumentation and expertise needed to perform RT-PCR prohibit its implementation at most public health settings in the US and abroad [10] . One approach to design NAT diagnostics without PCR amplification is to use a sandwich hybridization approach where target sequences are bound between two separate probes [19] . Normally one probe provides target segregation from the bulk solution (the surface probe), while the second probe imparts a measurable signal to the hybridization event (the reporter probe). The sandwich hybridization approach has been successfully implemented in a variety of nucleic acid sensing techniques, including: fluorescence imaging [20] , [21] , [22] , [23] , electrochemical detection [24] , [25] , [26] , template-mediated fluorescence activation [27] , [28] and surface-enhanced Raman scattering [29] . In most cases the requirement of two orthogonal binding events reduces background noise; however, the sensitivity of most sandwich assays is not as good as that achieved using a PCR-based method due to weak binding to the target or insufficient signal amplification. The aminoethylglycyl (aeg) peptide nucleic acid molecule (aegPNA) has nucleobases attached to a simple, non-natural polyamide backbone that consists of alternating ethylene diamine and glycine units ( Fig. 1a ) [30] . In general, aegPNA binds to complementary DNA and RNA sequences following Watson–Crick hydrogen bond pairing rules and forms duplex structures that are often more stable than duplexes of two nucleic acids ( Fig. 1b ) [31] , [32] . Since it is synthetic and does not occur in nature, aegPNA sequences are remarkably stable to degradation by proteases and nucleases [33] . Previously, we have shown that sequential introduction of cyclopentane groups into the PNA backbone (to create cyclopentane PNA) systematically enhances binding to target nucleic acid sequences ( Fig. 1c ) [34] , [35] , [36] , [37] . 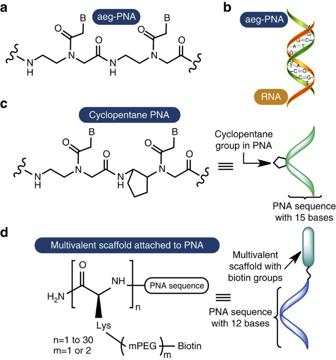Figure 1: Chemical structures and cartoon representations. (a) aegPNA showing two nucleobases (B=A, T, G or C). (b) aegPNA–RNA duplex. (c) Cyclopentane-modified PNA. The partial structure may be extended in either direction with additional aegPNA or cyclopentane PNA residues. (d) General strategy by which biotins are attached to the C-terminal of a PNA to create a multivalent scaffold with biotins. Figure 1: Chemical structures and cartoon representations. ( a ) aegPNA showing two nucleobases (B=A, T, G or C). ( b ) aegPNA–RNA duplex. ( c ) Cyclopentane-modified PNA. The partial structure may be extended in either direction with additional aegPNA or cyclopentane PNA residues. ( d ) General strategy by which biotins are attached to the C-terminal of a PNA to create a multivalent scaffold with biotins. Full size image In this manuscript we report the engineering principles to make a new type of RNA detection system that combines the accuracy of NAT with the practical convenience of enzyme-linked immunosorbent assay (ELISA) methodology. Key to the success of this merger is properly designed PNAs [30] , [31] , [32] that target HIV RNA sequences. By incorporating cyclopentanes into the surface PNA probe, we demonstrate that binding to the target RNA is significantly improved over aegPNA and subsequently improves nucleic acid detection. We have also designed a signal read-out system that can be coupled to the terminal end of a reporter PNA molecule to signal binding of a target RNA sequence. In this case, a unique chemical scaffold was developed to support the multivalent display of up to 30 biotin groups. The spacing of the biotins on the scaffold has been optimized to support assembly of multiple streptavidin-conjugated horseradish peroxidase enzymes around the terminal end of a PNA reporter probe (PNA-RP; Fig. 1d ). The assembly of this nanostructure upon PNA binding to target RNA sequences allows for dramatic signal amplification so that low levels of RNA are detectable. Proper combination of cyclopentanes in the surface PNA and multivalent biotins in the reporter PNA results in a synergistic improvement in detection for HIV RNA. Furthermore, we show that the optimized system can detect HIV RNA across a wide range of groups and clades of the virus, is compatible with detection of virus in human plasma, and that the results correlate with a current PCR standard of detection (COBAS Ampliprep v2.0; ref. 38 ). We also demonstrate that the enzymatic amplification system is robust (at least a 30 day shelf life at room temperature (RT)), that it is cost effective ($0.67 per well in a 96-well plate), and that the signal reporting on the amount of HIV can be determined either spectrophotometrically or with the naked eye. To abbreviate our detection method we have coined the term NAT-PELA, which stands for NAT–PNA Enzyme-Linked Assay. Sandwich setup for NAT-PELA In the current study, a sandwich hybridization assay using two PNAs is used to detect HIV RNA. The basic detection scheme is outlined in Fig. 2 . In this protocol, the first step is to attach a PNA surface probe (PNA-SP, 15 base sequence, see Supplementary Fig. 1 for all chemical structures and Supplementary Tables 1 and 2 for characterization) covalently via an amide bond to the plastic surface of a NUNC 96-well plate (i). PNA-RP (12 base sequence) is free in solution and contains biotin groups covalently attached to the C-terminal. The sequences of PNA-SP and PNA-RP are complementary to a 27-base sequence (5′- TTCTGCAGCTTCCTCATTGATGGTCTC -3′) that is part of HIV RNA in the gag region. If the target RNA is present, PNA-SP and PNA-RP both bind to their complementary sequences and a noncovalent complex of PNA-SP+PNA-RP+RNA is formed on the plastic surface (ii). The presentation of biotins from PNA-RP allows basic ELISA methodology to be used to amplify a signal for detection [39] . In this study, polyhorseradishperoxidase–streptavidin (pHRP–SA) is used in step iii to signal that the RNA target is present [40] . In this step, the streptavidin portion of pHRP–SA forms a strong complex with biotins attached to PNA-RP. Next, introduction of a substrate (tetramethylbenzidine (TMB) and peroxide) for the horseradishperoxidase enzyme part of pHRP–SA (step iv) results in oxidation of the tetramethylbenzidine to give products with blue colour [41] . The enzymatic oxidation reaction can be stopped by the addition of acid to afford yellow products (step v). Both the blue and yellow products can be quantified (at 652 nm and 450 nm, respectively) to show the level of RNA originally present. If the RNA target is not present in step ii, then PNA-RP is removed in subsequent wash steps, pHRP–SA cannot attach to the plastic surface, and no signal results when the tetramethylbenzidine solution is added. Tests for the stability of pHRP–SA showed that there is no loss in enzymatic activity for 30 days at RT ( Supplementary Fig. 2 ). 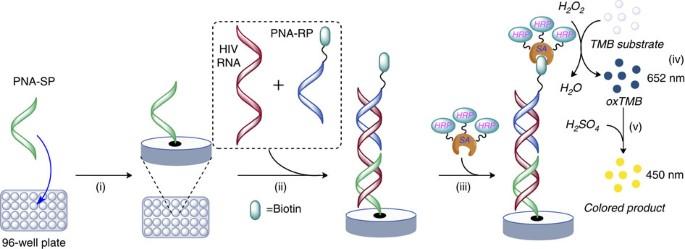Figure 2: General scheme for sandwich detection using a surface PNA (PNA-SP) and a reporter PNA (PNA-RP). (i) PNA-SP is covalently attached to the surface. (ii) If target HIV RNA is present, PNA-SP and PNA-RP both bind to their complementary sequences and a noncovalent complex is formed. In the absence of target RNA, PNA-RP is removed by subsequent washing steps. (iii) pHRP–SA is added. (iv) TMB is added and signal is monitored at 652 nm. (v) Enzymatic oxidation is stopped by the addition of sulphuric acid and the signal at 450 nm is measured. Figure 2: General scheme for sandwich detection using a surface PNA (PNA-SP) and a reporter PNA (PNA-RP). (i) PNA-SP is covalently attached to the surface. (ii) If target HIV RNA is present, PNA-SP and PNA-RP both bind to their complementary sequences and a noncovalent complex is formed. In the absence of target RNA, PNA-RP is removed by subsequent washing steps. (iii) pHRP–SA is added. (iv) TMB is added and signal is monitored at 652 nm. (v) Enzymatic oxidation is stopped by the addition of sulphuric acid and the signal at 450 nm is measured. Full size image Engineering, optimization and modelling of PNA-SP and PNA-RP A synthetic strand of HIV RNA with the 27-base target sequence was used to optimize the detection system. In all tests, the HIV RNA concentration in solution was varied and the data obtained at 652 nm and 450 nm were plotted as a function of absorbance versus time and absorbance versus concentration, respectively ( Fig. 3 ). The absorbance data at 450 nm, obtained after quenching of enzymatic oxidation with H 2 SO 4 , were plotted and subsequently fit to a four-parameter logistic curve to show the quantitative limits of detection ( Fig. 3d and Supplementary Fig. 3 ). To start, PNA-SP had no cyclopentane groups (PNA-SP0) ( Supplementary Fig. 1a ) and PNA-RP had one biotin (PNA-RP1) ( Supplementary Fig. 1f ). In this initial detection system, the lower limit of quantitative detection for the target RNA is in hundreds of millions (10 8 ) of molecules ( Table 1 and Supplementary Fig. 3a ). 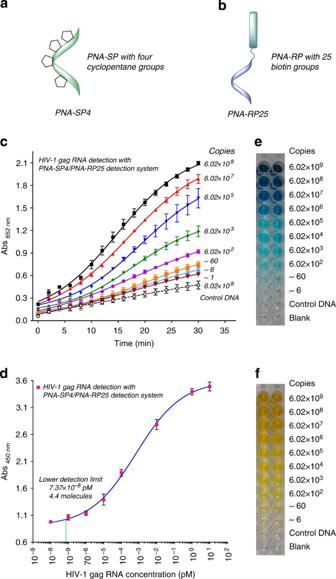Figure 3: Detection of the target HIV-1 gag RNA using the PNA-SP4/PNA-RP25 detection system. (a) Structure of PNA-SP4. (b) Structure of PNA-RP25. (c) Time-dependent absorbance (652 nm) changes upon analyzing different concentrations of HIV-1 gag RNA. (d) Signal response plots (absorbance at 450 nm versus concentration of HIV-1 gag RNA) obtained after quenching of enzymatic oxidation with H2SO4. The green line marks the minimal distinguishable differential concentration and represents the lowest limit of quantification. Forcandd, values represent the mean±s.d. of duplicate measurement (n=2) for each sample. (e,f) Photographs of the 96-well plate show the variation in colour intensity for HIV-1 gag RNA detection before (e) and after (f) quenching of enzymatic oxidation with H2SO4. Figure 3: Detection of the target HIV-1 gag RNA using the PNA-SP4/PNA-RP25 detection system. ( a ) Structure of PNA-SP4. ( b ) Structure of PNA-RP25. ( c ) Time-dependent absorbance (652 nm) changes upon analyzing different concentrations of HIV-1 gag RNA. ( d ) Signal response plots (absorbance at 450 nm versus concentration of HIV-1 gag RNA) obtained after quenching of enzymatic oxidation with H 2 SO 4 . The green line marks the minimal distinguishable differential concentration and represents the lowest limit of quantification. For c and d , values represent the mean±s.d. of duplicate measurement ( n =2) for each sample. ( e , f ) Photographs of the 96-well plate show the variation in colour intensity for HIV-1 gag RNA detection before ( e ) and after ( f ) quenching of enzymatic oxidation with H 2 SO 4 . Full size image Table 1 Modifications to PNA-SP and PNA-RP and effects on T m to complementary RNA and quantitative detection limit of detecting HIV target 27-base RNA (detection limits are presented in number of molecules of RNA). Full size table To improve this method so that it would be useful for clinical determination of HIV viral load, the limit of quantitative detection needed to be lowered to levels competitive with RT-PCR (which is ~20 molecules of RNA) [16] . Therefore, we explored the sequential incorporation of cyclopentane groups into PNA-SP ( Supplementary Fig. 1b–e ) and the incremental addition of biotin groups to the C-terminal of PNA-RP ( Supplementary Fig. 1g–m ). Additional cyclopentane groups in PNA-SP incrementally increases the binding affinity to the complementary RNA sequence ( Table 1 , SP1 to SP4, and Supplementary Table 2 ), and lowers the detection limit. Increasing the number of biotin groups on the end of PNA-RP enhances the signal intensity of the sandwich complex on the surface ( Fig. 4 ). Interestingly, there is a modest decrease in the binding of PNA-RP to its complementary RNA sequence as the number of biotins attached to the end increases ( Table 1 , RP1 to RP30, and Supplementary Table 2 ). This loss in binding, however, does not diminish the stability of the sandwich complex as the cyclopentanes in PNA-SP compensate for any loss in stability ( Supplementary Table 2 ). Attempts to incorporate cyclopentane groups into PNA-RP were not successful when large numbers of biotin groups were required. Quantitative detection limits were determined for every combination of PNA-SP and PNA-RP, and the results are presented in Table 1 . Both types of modifications work together to lower the limit of RNA detection. In the optimal system, PNA-SP with four cyclopentane groups ( Fig. 3a ) and PNA-RP with 25 biotin groups ( Fig. 3b ) was sufficient to detect HIV RNA in a region that would be competitive with PCR diagnostics ( Fig. 3c,d ), and the detection of 60 copies could also be observed visually ( Fig. 3e,f ). Additional biotins did not further enhance detection (PNA-RP30, Supplementary Fig. 1m and Table 1 ). Notably, these engineering principles were able to improve detection of the target RNA by about 8 orders of magnitude from the original system (PNA-SP0 and PNA-RP1). 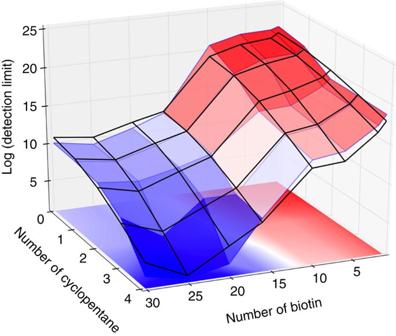Figure 4: Detection limits as a function of biotin and cyclopentane. Coloured regions: three-dimensional representation ofTable 1. Detection limits are represented on thez-axis as the log10of the number of molecules of RNA, versus the number of cyclopentanes in PNA-SP and number of biotins in PNA-RP. The red colour indicates higher detection limits, while blue represents favourable, lower detection limits. The same data is projected as a contour map underneath. Black wireframe: the model equation derived from PCA (RMSD 0.67 relative to the experimental data) as described in Principle Component Analysis model in the Methods section. Figure 4: Detection limits as a function of biotin and cyclopentane. Coloured regions: three-dimensional representation of Table 1 . Detection limits are represented on the z -axis as the log 10 of the number of molecules of RNA, versus the number of cyclopentanes in PNA-SP and number of biotins in PNA-RP. The red colour indicates higher detection limits, while blue represents favourable, lower detection limits. The same data is projected as a contour map underneath. Black wireframe: the model equation derived from PCA (RMSD 0.67 relative to the experimental data) as described in Principle Component Analysis model in the Methods section. Full size image A model was developed to explain the relative contributions of adding cyclopentanes and biotins into PNA-SP and PNA-RP. As input, the logs of the detection limits from Table 1 were represented on a three-dimensional plot (coloured regions in Fig. 4 ). Attempting to fit a plane to the detection limits resulted in a poor fit, with a root-mean-square deviation (RMSD) of 1.9. This implies that a simple linear relationship between detection limits, cyclopentanes and biotins does not exist ( Supplementary Fig. 4 ). Considering that PNA-SP should retain RNA on the surface and directly influence the final concentration for detection, a simple model was developed where the detection limit is a function of the cyclopentanes plus a separable product of cyclopentane and biotin functions. This is represented by f ( x , y )= h 1 ( x )+ h 2 ( x ) h 3 ( y ), where f ( x , y ) is the log of the detection limit, x is the number of cyclopentanes in PNA-SP, and y is the number of biotins in PNA-RP. The form of our model is especially amenable to Principle Component Analysis (PCA) [42] . In this approach, a series of orthogonal vectors are fit to the data set with the goal of identifying a set of principle vectors that best represent the data with minimal variance. Prior to PCA, the data is mean centred with respect to cyclopentanes, h 1 ( x ). By retaining only the largest component, the principle component vector and its associated loading vector are h 2 ( x ) and h 3 ( y ), respectively. This model accounts for 90% of the variance of the original data (RMSD 0.67). The dark lines in Fig. 4 represent the model overlaid with the original data in colour. This decomposition was examined to gauge the contributions of cyclopentanes and biotins to the detection limit. As shown in Supplementary Fig. 5b , the monotonic increase in cyclopentane groups lowers detection ( h 2 ). For biotin there is a general trend that adding more biotins improves detection, but the functional form of improvement is more complex ( h 3 ). As shown in Supplementary Fig. 5c , additional biotins can lower detection limits at specific intervals of biotins (such as those around 6 and 25 biotins) but in other ranges there is no improvement or even slight worsening of the detection limit (such as ~16 biotins). Detection of HIV in plasma The optimized PNAs (PNA-SP4 and PNA-RP25) were used to detect full length HIV RNA derived from samples where the virus was added into human plasma. For these sets of experiments, RNA extraction from the HIV-positive plasma samples was performed using the commercial reagent RNAzolRT following the manufacturer’s procedures [43] . To determine whether the PNA probes could detect different genetic variants of HIV, seven different clades and two groups of the virus were tested under the same procedures. For all examples, the NAT-PELA system was able to quantify virus at levels (around 20 molecules of RNA) consistent with clinically useful levels ( Fig. 5 ; Supplementary Fig. 6 ). 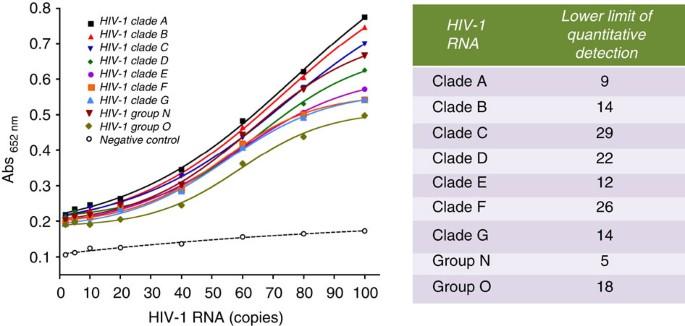Figure 5: Detection of seven different subtypes and two different groups of HIV-1 RNA using the PNA-SP4/PNA-RP25 detection system. The plot shows the signal response (absorbance at 652 nm versus concentration of HIV-1 RNA) obtained after 30 min. The table shows the calculated minimal distinguishable differential concentration, which represents the lowest limit of quantification. Each value in the table represents the smallest number of HIV-1 RNA molecules that could be detected based on the curve fit to the absorbance data versus RNA concentration at 90% confidence intervals. The negative control represents the signal obtained when virus-free plasma is subjected to the same NAT-PELA detection protocol. Figure 5: Detection of seven different subtypes and two different groups of HIV-1 RNA using the PNA-SP4/PNA-RP25 detection system. The plot shows the signal response (absorbance at 652 nm versus concentration of HIV-1 RNA) obtained after 30 min. The table shows the calculated minimal distinguishable differential concentration, which represents the lowest limit of quantification. Each value in the table represents the smallest number of HIV-1 RNA molecules that could be detected based on the curve fit to the absorbance data versus RNA concentration at 90% confidence intervals. The negative control represents the signal obtained when virus-free plasma is subjected to the same NAT-PELA detection protocol. Full size image Titration curve for NAT-PELA with HIV-spiked plasma samples To prepare NAT-PELA for detection of patient samples, a titration curve was determined using different concentrations of the virus. For these experiments, clade B HIV virus was spiked into human plasma and then subsequently diluted with additional human plasma to simulate a range of clinical concentrations for the virus. Each sample was then tested by both PCR (using COBAS Ampliprep v2.0; ref. 38 ) and by the NAT-PELA procedure. For the PCR tests, plasma samples were directly processed by the instrumentation. For the NAT-PELA tests, RNA extraction using RNAzolRT was performed for each plasma sample with a different HIV concentration [43] . The titration curve of NAT-PELA is shown in Supplementary Fig. 7 . The quantitative values of virus in this experiment are determined by PCR. This experiment demonstrated that NAT-PELA provides clear signals over a range of HIV concentrations from 20 to 30,000 copies of HIV per ml of plasma. Detection of HIV in patient samples by NAT-PELA and PCR Finally, NAT-PELA was used to detect HIV in 20 plasma samples, each one from a different HIV-positive patient, representing a concentration range from 100 to 25,000 copies per ml of plasma. For each patient sample, there was sufficient volume for two PCR tests using the COBAS Ampliprep instrumentation and for one test by NAT-PELA. Processing of all samples was performed using the same protocol previously mentioned for the titration curve. For every HIV-positive patient sample, NAT-PELA showed higher absorbance signals over the control plasma samples that were HIV negative. The variation in signal intensity for NAT-PELA changes with concentration of the virus ( Fig. 6 ), with the greatest change in signal occurring at the concentrations that are below ~1,500 copies of virus per ml of plasma ( Fig. 6c , full data in Supplementary Fig. 8 and Supplementary Table 3 ). The NAT-PELA data for the samples with low viral loads showed a strong linear correlation with change in PCR-determined viral load (coefficient of determination R 2 =0.93, Pearson product-moment correlation P <0.01). At viral loads greater than 2,000 copies per ml of plasma, NAT-PELA shows very strong absorbance readings that are >1, which results in a loss of linear correlation with HIV concentration due to the high absorbance of these samples. Therefore, NAT-PELA is able to quantify HIV viral loads at 1,500 copies per ml of plasma or lower, and can be used qualitatively to signal higher viral loads. 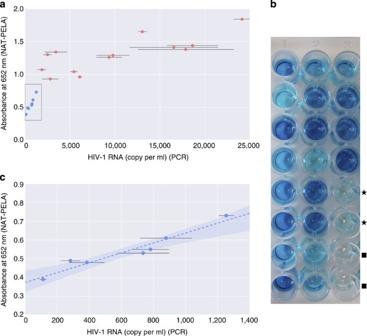Figure 6: HIV-1 quantification of patient samples with NAT-PELA (using PNA-SP4 and PNA-RP25) and PCR. (a) NAT-PELA data for all patient samples. Boxed region shows the samples with HIV viral loads <1,500 copies per ml of plasma. (b) Photograph of the 96-well plate, showing the variation in color intensity for HIV-1 RNA detection in patient samples by NAT-PELA. The wells designated by the star (*) are the results of using HIV-negative plasma, the wells designated by the square (▪) are controls without RNA target. (c) Linear correlation between NAT-PELA and PCR viral load over 100 to 1,500 copies of HIV per ml of plasma. Linear fit to the data (R2=0.93) with the shaded region representing a bootstrapped 95% confidence interval. There is a strong linear correlation of NAT-PELA signal with changes in HIV viral load (Pearson coefficientP<0.01). Figure 6: HIV-1 quantification of patient samples with NAT-PELA (using PNA-SP4 and PNA-RP25) and PCR. ( a ) NAT-PELA data for all patient samples. Boxed region shows the samples with HIV viral loads <1,500 copies per ml of plasma. ( b ) Photograph of the 96-well plate, showing the variation in color intensity for HIV-1 RNA detection in patient samples by NAT-PELA. The wells designated by the star (*) are the results of using HIV-negative plasma, the wells designated by the square (▪) are controls without RNA target. ( c ) Linear correlation between NAT-PELA and PCR viral load over 100 to 1,500 copies of HIV per ml of plasma. Linear fit to the data ( R 2 =0.93) with the shaded region representing a bootstrapped 95% confidence interval. There is a strong linear correlation of NAT-PELA signal with changes in HIV viral load (Pearson coefficient P <0.01). Full size image Antibody-based diagnostics using ELISA can provide a rapid readout of infection status as these tests can be coupled to automated engineering platforms that simplify routine testing [44] . Developing highly specific antibodies for biomarkers of diseases is crucial for any ELISA-based technology to be successful. We propose that NAT-PELA should similarly benefit NAT because automated ELISA technology could be readily adapted to use the PNA probes presented in this manuscript. In the same way that antibodies must be properly engineered for any ELISA-based assay, we find that PNAs also must be carefully designed for NAT-PELA to be successful and competitive with PCR. In the area of HIV diagnostics, the viral load of an infected individual must be routinely determined throughout therapeutic treatment to make certain that any medication maintains the virus at low levels [45] . The NAT-PELA protocol we have developed with PNA-SP4 and PNA-RP25 has sufficient sensitivity to detect and quantify HIV in patient plasma within a concentration range that would be useful for assisting with the selection of appropriate therapy. The same system may also be used to qualitatively signal a high level of virus in excess of 2,000 copies per ml of plasma. Samples that are too concentrated to be quantified could be diluted to a lower concentration that is within the range for quantification by the NAT-PELA system. While PCR-based methods to determine HIV viral loads are routine, new methods based on NAT-PELA may offer a more cost-effective alternative. In our laboratory, the reagent cost to perform one assay in a single well of a 96-well plate is about $0.67 ( Supplementary Table 4 ). This cost includes the synthetic costs to make PNA-SP4 and PNA-RP25 as well as all additional reagents and buffers, but it does not include costs to purchase any instrumentation or any labour costs to perform the assay. The methods we present in this manuscript provide the basic concepts to design PNA probes for an automated NAT-PELA system for monitoring HIV or any other RNA-based markers of disease. Reagents and materials All t -butyloxycarbonyl (Boc)- and 9-fluorenylmethoxycarbonyl (Fmoc)-PNA monomers were purchased from PolyOrg, Inc. (Leominster, MA, USA); cyclopentane T and A PNA monomer was made following previously published procedures [37] . Acetonitrile, acetic anhydride (Ac 2 O), pyridine, thioanisole, bovine serum albumin, dichloromethane (DCM), N,N-di-isopropylethylamine (DIEA), N,N-dimethylformamide (DMF), EDTA, diethyl ether (Et 2 O), Kaiser test reagents, m-cresol, Na 2 CO 3 , N -methyl-2-pyrrolidinone (NMP), piperidine, sealing film for multi-well plates, trifluoroacetic acid (TFA), trifluoromethanesulfonic acid, polysorbate 20 (Tween 20) and single-stranded salmon sperm DNA were purchased from Sigma-Aldrich (St Louis, MO, USA). 1-Step Ultra-TMB, 96-well Nunc Immobilizer Amino plates, pHRP–SA was obtained from Thermo Scientific (Fairlawn, NJ, USA). RNA and DNA oligomers were ordered from IDT (Coralville, IA, USA). PBS was purchased from Quality Biological (Gaithersburg, MD, USA). High purity water (18 MΩ) was generated from a Millipore (Billerica, MA, USA) Milli-Q water system. Boc-8-amino-3,6-dioxaoctanoic acid (Boc-mPEG-OH), Fmoc-8-amino-3,6-dioxaoctanoic acid (Fmoc-mPEG-OH) and Boc-11-amino-3,6,9-trioxaundecanoic acid (Boc-mPEG3-OH) were purchased from Peptides International (Louisville, KY, USA). O -benzatriazole- N , N , N ′, N ′-tetramethylammoniumhexafluorophosphate (HBTU), Fmoc-Lys(Boc)-OH, H-Lys-OH·HCl and methyl-benzhydrylamine (MBHA) resin were purchased from Advanced Chemtech (Louisville, KY, USA). H 2 SO 4 was purchased from EMD Chemicals (Gibbstown, NJ, USA). RNAzolRT was obtained from Molecular Research Center, Inc. (Cincinnati, OH, USA). Resin downloading protocol MBHA resin was downloaded from 0.3 to 0.1 mmol g −1 using Boc-Lys(2-Cl-Z)-OH or Boc-G(Z)-OH. The MBHA resin (1.0 g) was swelled with DCM for 1 h in a peptide synthesis vessel. The following solutions were prepared: (a) 0.4 M Boc-Lys(2-Cl-Z)-OH in NMP, or 0.4 M Boc-G(Z)-OH in NMP, (b) 0.2 M HBTU in DMF and (c) 0.5 M DIEA in NMP. Next, 450 μl of solution a, 460 μl of solution c and 1.59 ml NMP were combined and mixed to make solution 1. Then, 550 μl of solution b were diluted with NMP (1.95 ml) to make solution 2. Solutions 1 and 2 were combined and pre-mixed for ~30 s before adding to the drained, swelled resin. The resin/coupling mixture was agitated for 1 h before draining and washing with DMF (4 × ), DCM (4 × ), 5% DIEA in DCM (1 × ~30 s) and finally DCM (4 × ). Any remaining active sites were capped using capping cocktail (1:25:25 Ac 2 O:NMP:pyridine) for 20 min. The reaction was drained and rinsed with DMF (3 × ) and DCM (3 × ). The progress of the capping was followed by a qualitative Kaiser test. If the test was positive, the resin was resubmitted to capping. After a negative test for primary amines, the resin was washed with DCM (3 × ) and dried under vacuum for 30–60 min and then stored in a dessicator. General method for PNA synthesis PNAs were prepared on 5 μmol scale using either Boc- or Fmoc-solid phase peptide synthesis protocols on an Applied Biosystems 433a automated peptide synthesizer with HBTU as the amide-forming reagent. All PNA-SP were synthesized on Boc-G(Z)-OH downloaded MBHA resin, and all PNA-RP were synthesized on Boc-Lys(2-Cl-Z)-OH downloaded MBHA resin. Cleavage and recovery of crude PNA from resin The resin, in a peptide synthesis vessel, was first washed with TFA (2 × for 4 min). To the drained resin, cleavage cocktail (1.5 ml, 900 μl:300 μl:150 μl:150 μl TFA/trifluoromethanesulfonic acid/thioanisole/m-cresol), cooled over ice, was added and reacted for 1 h. The cleavage mixture was collected in a glass vial using N 2 pressure to drain the vessel. The resin was resubmitted to fresh cleavage cocktail and cleaved for 1 h, and was drained into the first cleavage fraction. The volatiles were removed by flowing dry N 2 over the solution to produce a yellow-brown oil. Approximately 10 ml of Et 2 O was added to the cleavage oil to create a suspended white precipitate. The suspension was partitioned into five 2 ml microcentrifuge tubes and chilled over dry ice for 10 min. The tubes were centrifuged at 12,000 r.p.m. for 40 s to produce a white pellet. Et 2 O was carefully decanted, leaving the white crude PNA solid. Further washing was performed by adding ~1.6 ml of Et 2 O to each tube, mixing to resuspend the precipitate, then chilling on dry ice for 5 min. Following centrifugation and decanting, the washes were repeated twice without dry ice. After the final wash, the white precipitate was dried by carefully passing a stream of dry N 2 over the crude PNA. Purification of crude PNA and characterization Purification was performed on an Agilent (Santa Clara, CA) 1200 Series RP-HPLC with automatic fraction collection using ultraviolet detection at 260 nm. Waters (Milford, MA, USA) XBridge C18 (10 × 250 mm, 5 μm) columns were used in conjunction with Solvents A and B. Solvent A was 0.05% TFA in water and Solvent B consisted of 90% acetonitrile in water. PNA HPLC isolates were characterized using electrospray ionization-mass spectrometry on a Waters/Micromass LCT Premier time-of-flight mass spectrometer. The instrument was operated in W-mode at a nominal resolution of 10,000. The electrospray capillary voltage was 2 kV and the sample cone voltage was 60 V. The desolvation temperature was 275 °C and the desolvation gas was N 2 with a flow of 300 l h −1 . Accurate masses were obtained using the internal reference standard method. The sample was introduced into the mass spectrometer via the direct loop injection method. Deconvolution of multiply charged ions was performed with MaxEnt I. All PNA oligomers gave molecular ions consistent with the calculated theoretical product values ( Supplementary Table 1 ). Thermal melting analysis Ultraviolet concentration was determined by adding 4 μl of RNA solution to 196 μl milli-Q water. If the signal was too intense the concentration was diluted by adding 198 μl of water to 2 μl of the original RNA solution. Water was blanked against the background at 80 °C on an Agilent 8453 UV/Vis spectrometer equipped with an Agilent 89090A Peltier temperature controller and a computer interface. Then the unknown solution was added to the quartz cell (Helma) and vigorously shaken, replaced in the spectrophotometer and the absorbance was read at 260 nm. The mixing and reading was repeated three times. Values were converted to concentration, based on average absorbance. After initial measurement by ultraviolet, the concentration was determined based on appropriate ε 260 nm (calculated on nearest neighbour approximation for PNA or provided by IDT or Thermo Scientific for oligonucleotides) and then used from that point forward for additional experiments. Thermal melting experiments were performed by preparing 2 μM oligonucleotide solution in 1 × PBS. Experiments traversed from 90 to 20 °C and back to 90 °C at 1 °C intervals while monitoring at 260 nm. An equilibration of 60 s at each temperature measurement step before readings was employed. Cooling and heating profiles were generated for each run with duplicates for each. The T m (melting temperature) for duplexes was determined using the maximum first derivative of the cooling and heating curves, then taken as an average of both runs. Buffers for NAT-PELA Blocking buffer (BLB): 2% bovine serum albumin, 25 mM tris(hydroxymethyl) aminomethane (Tris), 150 mM NaCl, 0.05% TWEEN 20, 0.1 mM EDTA, pH 7.4; BLBs: BLB with 0.1 μg ml −1 single-stranded salmon sperm DNA; Capping solution (CAP): 25 mM Lys, 10 mM NaH 2 PO 4 , 100 mM NaCl, 0.1 mM EDTA, pH 8.0; immobilization buffer: 100 mM Na 2 CO 3 , pH 9.6; 1 × PBS: PBS, 9.0 g l −1 NaCl, 144 mg l −1 KH 2 PO 4 , 795 mg l −1 Na 2 HPO 4 , pH 7.4; 1 × PBST: 1 × PBS with 0.05% Tween 20. Plate preparation PNA-SP was dissolved in immobilization buffer (1.0 μM) and a volume of 100 μl was added to each well of the plate. Blank wells were left untouched throughout the process to blank against the plate. The plate was sealed with sealing tape for multi-well plates and agitated on a plate shaker (600–700 r.p.m.) for 2 h at RT. Then 50 μl of CAP was added to modified wells to give a final volume of 150 μl. This was again agitated at RT on a plate shaker for 30 min. Modified wells were then aspirated and washed four times with 300 μl of 1 × PBST and four times with 1 × PBS. A final addition of 250 μl of 1 × PBS was used to store the wells until used in experiments. When the assay was ready to be performed, the 1 × PBS was removed by aspiration and 200 μl BLBs was added to the wells. The plate was sealed and incubated with shaking for 30 min at 37 °C, the wells were immediately aspirated and ready for sample addition. Preparation of synthetic HIV-1 gag RNA samples All samples were prepared in glass vials. Synthetic RNA was ordered from IDT. The final volume for all samples used for RNA detection was 600 μl. Each of these samples had the PNA-RP concentration fixed at 15 nM. The specific concentration of the target RNA for detection was prepared by a serial dilution of a stock 50 nM solution of the RNA target in 1 × PBS buffer prepared from the commercial RNA. The initial (and highest concentration) RNA sample for detection was the first sample made, using the desired amount of RNA from the 50 nM stock solution and diluting with a solution of the reporter probe (PNA-RP, 15 nM) in 1 × PBS buffer. To dilute further from the initial RNA detection sample, a desired volume of RNA solution was removed and further diluted with the 15 nM reporter probe solution in 1 × PBS buffer. For example, to dilute an initial 450 pM RNA sample solution by three times, 200 μl of the initial RNA sample solution was removed and added to 400 μl of 15 nM reporter probe solution in 1 × PBS buffer to give a final RNA concentration of 150 pM. Once the final RNA concentration was obtained after dilution, the samples were heated to 95 °C in a sand bath for 5 min and then snap-cooled by placing the vials directly into an ice bath for 5 min. Then, the samples were directly used for RNA detection by removing 100 μl of each sample and individually adding the RNA solution to one well on the prepared 96-well plate (using a 100 μl pipettor). To construct a concentration-dependent response curve, 10 different RNA concentrations were prepared and each concentration was prepared in duplicate. Two wells of each plate were dedicated to the detection of one RNA concentration. After the samples were added to the wells, the plate was sealed and incubated with shaking at 37 °C for 3 h. Each well was aspirated following incubation and then washed with 300 μl of 1 × PBST four times followed by 300 μl of 1 × PBS four times. HIV-1 RNA extraction by RNAzolRT Analysis of patient samples was approved by the Office of Human Subjects Research at NIH (National Institutes of Health). Virus was isolated from peripheral blood mononuclear cell samples of HIV-1-positive individuals infected with nine different HIV-1 subtypes (Clades A, B, C, D, E, F, G, and Groups N and O). The culture supernatants were harvested and spiked in Base matrix. Viral loads were measured by the Abbott RealTime HIV-1 system (Abbott Molecular Inc. Des Plaines, IL, USA). One plasma sample from an HIV-1-negative individual was also included as a negative control. For extraction of HIV-1 RNA using RNAzolRT, 400 μl of plasma was mixed with 1 ml of RNAzolRT reagent followed by the addition of 200 μl RNAase free water and mixed well. Samples were incubated at RT for 15 min and centrifuged at 12,000 g , 4 °C for another 15 min. The upper layer was removed (~1500 μl) and an equal volume of isopropanol was added and mixed well by tilting tubes. The tubes were left at RT for 15 min after which they were centrifuged at 12,000 g for 15 min, aspirated and washed with 70% ethanol twice. The pellets were dried and dissolved in 50 μl of RNAase free water. Correlation of NAT-PELA with RT-PCR HIV-1-positive plasma (Clade B) with viral loads of 1.5 × 10 9 copies per ml, stored at −80 °C, was diluted to 10,000, 5,000, 1,000, 500, 100, 50 and 10 copies per ml in HIV-1-negative plasma (base matrix). A total of 6 ml volume was prepared for each concentration, and divided into six tubes with 1 ml each. For each concentration, RNA extraction using RNAzolRT was independently performed on three 1 ml samples and the isolated RNA from each sample was subsequently used in the NAT-PELA assay. The remaining three 1 ml samples at the same concentration were subjected to the COBAS AmpliPrep/COBAS TaqMan HIV-1 Test (Roche Molecular Systems, Inc., Branchburg, NJ, USA). HIV-1 RNA detection in patient plasma samples Twenty plasma samples collected from 20 different HIV-positive patients were each tested by NAT-PELA and RT-PCR. Each plasma sample consisted of 3 ml total volume that was divided into three tubes with 1 ml of plasma in each tube. For each patient sample, one of the 1 ml tubes was tested using NAT-PELA (where the RNA was extracted using RNAzolRT), and the other two 1 ml tubes for each patient sample were tested using the COBAS AmpliPrep/COBAS TaqMan HIV-1 Test. To exclude the possibility of biased results due to non-specific interactions, two HIV-negative plasma samples were also included. NAT-PELA protocol The wells were incubated with 200 μl of BLB. The plate was sealed and shaken at 37 °C for 30 min. Wells were then aspirated, following by addition of 100 μl of 0.1 μg ml −1 pHRP–SA in BLB. The plate was sealed and incubated for 20 min at RT before aspirating. The wells were aspirated and followed a washing procedure that consisted of 300 μl of four times of 1 × PBST and four times of 1 × PBS. NAT-PELA readout Following washes, 100 μl 1-Step Ultra TMB solution was added via a multichannel pipette to facilitate nearly simultaneous initial starting points for all wells. The plate was immediately placed in a Molecular Devices (Sunnyvale, CA, USA) SpectraMax M5 multi-mode microplate reader and monitored at 652 nm over the course of 30 min at RT. The plate was then removed, followed by addition of 50 μl 2 M H 2 SO 4 and mixed by hand for 10 s to quench the enzyme reaction. The plate was then returned to the plate reader and a final reading at 450 nm was performed. Plates were sealed with a film following reading and placed in the refrigerator. Analysis of NAT-PELA results Analysis of absorbance (652 nm) kinetics . The absorbance was monitored at 2 min intervals over 30 min (16 pts) at each concentration of target nucleic acid. The absorbance at 652 nm was plotted versus time to give the kinetic curve for each concentration using Prism 4.0 software ( Fig. 3c ), from which we can clearly see the qualitative detection limit. Nonlinear regression analysis of quenched assay results. The protocol employing quenched TMB product that used end point absorbance values at 450 nm was used as a response value and plotted with respect to target nucleic acid concentration using Prism 4.0 software. The limits of quantitation for the HIV-1 RNA were determined using the 4-PL models with Prism 4.0 software by calculating the upper limit of the zero analyte concentration parameter error using a 90% confidence interval. These values provide a limit that is distinguishable from background noise with 96% certainty (Minimal distinguishable differential concentration). The resulting fits are graphically represented in Supplementary Fig. 3 , and the quantitative detection limits are listed in Table 1 . Four-PL model equation: y = A +(( D − A )/(1+10 (log C − x ) B )), where A is the response at a concentration of zero (baseline); B is the slope factor; C is the inflection point (IC50); D is the response at infinite concentration; Y is the response; X is the analyte concentration. Enzyme stability study The pHRP–SA stability was determined by incubating the enzyme at RT for different times. Ten millilitres of 0.1 μg ml −1 pHRP–SA was prepared in BLB and was incubated at RT for 0, 1, 2, 4, 6, 8, 10, 15, 20, 25, 30, 35, 40, 45, 50, 55 and 60 days. Aliquots were withdrawn at each time point to test the remaining activity by SP0/ RP1/HIV-1 gag synthetic 27-nucleobase single-stranded DNA at standard conditions as described above, the target HIV-1 gag DNA concentration is 100 pM. The fresh prepared enzyme was considered to be a control and was assumed to have 100% activity. PCA model The data in Table 1 represent the detection limits as a function of the number of cyclopentanes in PNA-SP and biotins in PNA-RP. Attempts were made to develop a qualitative model that explains the dependence of the detection limits on these two variables. A simple linear response, where the dependence of the detection limit is fit to a simple plane, does not adequately explain the data ( Supplementary Fig. 5 ). We next recast the data in terms of a function, f( x , y ), where f is the detection limit, x is the number of cyclopentanes in PNA-SP and y is the number of biotins in PNA-RP. We hypothesize that the interaction of the two variables is largely separable, in which case the following equation: f ( x , y )= h 1 ( x )+ h 2 ( x ) h 3 ( y ) should be true where h 1 ( x )=< f ( x , y )> x is the signal at a fixed value of cyclopentane, averaged over all the observations of biotin. This formulation naturally leads to a decomposition with PCA. This is a classic algorithmic tool to reduce multidimensional data sets into a series of orthogonal vectors designed to maximize the explained variance in each direction. Ideally, after the analysis, the data can be reproduced with a subset of these principle component vectors. In addition, if the largest principal component is relatively dominant to the others, its components can give physical insight to the contributions of individual components (in this case the addition of cyclopentane groups and biotin groups). We find that a significant fraction of the variance in Table 1 can be explained using only the largest principal component from the PCA. To perform the PCA, the first consideration is that the measured data points of Table 1 are not on a regular grid. To remove undue weight on closely centred observations, a linearly interpolated matrix at 500 regularly spaced intervals was constructed between the data range. We perform PCA on this matrix by first subtracting the mean for each row and taking the singular value decomposition of the remaining matrix F , so that: where D is a square diagonal matrix of singular values and the columns of U and W are the left and right singular vectors. A subset of the L largest principal components can be constructed by noting T L =U L D L =FW L . The columns of U , multiplied by the magnitude of the associated element of the diagonal matrix, U i D ii are known as the principal components, while the columns of W are known as the loading vectors. The principal components are a linear combination of the input data while the loading vectors associate a weight to each variable in this linear combination. We find that the largest principal component can explain 90% of the variance of the data. An illustration of the signal projected using only the largest component is shown in Fig. 4 . The directions of the principal components and the mean values, h 1 ( x ), h 2 ( x ) and h 3 ( y ) are shown in Supplementary Fig. 5 . It is evident that the effect of cyclopentane gives a favourable monotonic decrease in the signal detection limit. The effect of adding more biotins, while generally favourable, shows a more complicated contribution to the detection limit. How to cite this article: Zhao, C. et al . Quantification of plasma HIV RNA using chemically engineered peptide nucleic acids. Nat. Commun. 5:5079 doi: 10.1038/ncomms6079 (2014).